Massive outbreaks ofNoctiluca scintillansblooms in the Arabian Sea due to spread of hypoxia In the last decade, the northern Arabian Sea has witnessed a radical shift in the composition of winter phytoplankton blooms, which previously comprised mainly of diatoms, the unicellular, siliceous photosynthetic organisms favoured by nutrient-enriched waters from convective mixing. These trophically important diatom blooms have been replaced by widespread blooms of a large, green dinoflagellate, Noctiluca scintillans , which combines carbon fixation from its chlorophyll-containing endosymbiont with ingestion of prey. Here, we report that these massive outbreaks of N. scintillans during winter are being facilitated by an unprecedented influx of oxygen deficient waters into the euphotic zone and by the extraordinary ability of its endosymbiont Pedinomonas noctilucae to fix carbon more efficiently than other phytoplankton under hypoxic conditions. We contend that N. scintillans blooms could disrupt the traditional diatom-sustained food chain to the detriment of regional fisheries and long-term health of an ecosystem supporting a coastal population of nearly 120 million people. The multi-disciplinary Joint Global Ocean Flux Study (JGOFS) [1] , [2] programme in the Arabian Sea (1994–1996) showed that monsoonal winds and their reversal from southwesterly in summer to northeasterly in winter fertilize the normally nutrient-depleted euphotic zone and produce the greatest seasonal extremes of phytoplankton biomass, carbon fixation and carbon flux observed in any of the world’s oceans. Carbon cycling and export from the ocean surface were found to be largely a function of changes in the food web structure driven by monsoonal alterations in nutrient concentrations [1] . In general, before, and following the winter monsoon, both periods of low nutrient concentrations and carbon export, surface waters are dominated by autotrophic picoplankton Prochlorococcus and Synechococcus [1] . In contrast, during summer and winter monsoons, higher primary production and carbon export are coincident with large diatom blooms [1] , [3] fuelled by elevated nutrient concentrations from summer coastal upwelling [1] and winter convective mixing [3] , respectively. Since the end of the JGOFS programme, there have been no large-scale field campaigns in the Arabian Sea. Most contemporary estimates of phytoplankton biomass (estimated as Chlorophyll a , Chl a ), productivity and carbon cycling have come from satellite-based observations [4] , [5] or coupled biophysical models [6] . Beginning in 2003, our field studies have provided large datasets of the taxonomic structure [4] , [5] , [7] of winter phytoplankton communities which show a drastic shift from diatom-dominated blooms to thick and widespread blooms composed primarily of the green dinoflagellate, N. scintillans. Unlike the red form reported mostly in temperate coastal waters worldwide [8] , this Arabian Sea N. scintillans is green because of its large endosymbiotic population of free-swimming cells of Pedinomonas noctilucae (Class Prasinophyceae, Division Chlorophyta) [9] , [10] ( Fig. 1a–c , Supplementary Movie 1 ). It is also large (0.5–1.2 mm; Fig. 1a ) compared with its temperate counterpart [9] . Before the appearance of large-scale green N. scintillans blooms in the open ocean waters of Arabian Sea in winter, the green N. scintillans was observed only sporadically, confined to coastal waters along the west coast of India [11] , [12] . Conversely, the heterotrophic red N. scintillans that contains no endosymbionts and survives solely by grazing was seen confined [13] , [14] , [15] to the southwest coast of India, in summer when the region experiences upwelling [16] . Blooms of the red N. scintillans were also observed in the Gulf of Oman every year between January and May since 1988 (ref. 17 ) but from the early 1990s the green variety is also being seen with increasing intensity with peaks in both summer and in winter [18] . 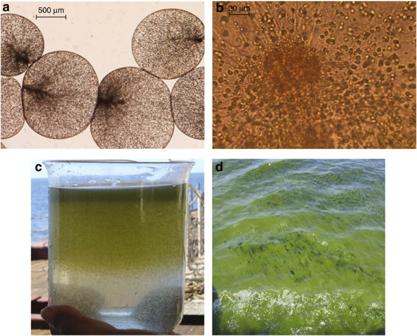Figure 1:N. scintillanswith endosymbionts and as a bloom in the Arabian Sea. (a) Single cells ofN. scintillanswith the endosymbiontP. noctilucaecollected on 17 February 2009 at St 6 (20.9° N Lat., 66.17°E Long.). (b) Close-up ofN. scintillanswith endosymbiontP. noctilucaeand ingested diatoms. (c)N. scintillansin a beaker showing the density of the bloom. (d) Thick surface bloom ofN. scintillansin the Arabian Sea on 17 February 2009. Figure 1: N. scintillans with endosymbionts and as a bloom in the Arabian Sea. ( a ) Single cells of N. scintillans with the endosymbiont P. noctilucae collected on 17 February 2009 at St 6 (20.9° N Lat., 66.17°E Long.). ( b ) Close-up of N. scintillans with endosymbiont P. noctilucae and ingested diatoms. ( c ) N. scintillans in a beaker showing the density of the bloom. ( d ) Thick surface bloom of N. scintillans in the Arabian Sea on 17 February 2009. Full size image From 2009 to 2011, we conducted programmatically focussed cruises with two goals: to determine the causative factors for the recent outbreaks of the green N. scintillans blooms in the open Arabian Sea and to assess the potential consequences of these basin-wide blooms for its ecosystem. A large archive of shipboard datasets together with shipboard experiments conducted for 2 years are utilized to support our conclusions that the massive outbreaks of the green N. scintillans are being promoted by the recent appearance of hypoxic waters at the sea surface. Switchover in dominant species of winter phytoplankton bloom Since they were first observed in the open ocean waters of the Arabian Sea in the early, 2000s, blooms of the green N. scintillans , now occur every year with predictable regularity from January to March. The basin-wide expanse of the blooms over the entire Arabian Sea and the consistency of their appearance each year are captured in the February ocean colour Aqua-MODIS images for three consecutive years (2009–2011; Fig. 2a–c ). Within a bloom, N. scintillans concentrations average about 1,200 cells l −1 , but can reach as high as 9,600 cells l −1 as recorded during our cruise of February 2009 when thick green blooms covered the sea surface ( Fig. 1d ). When in peak bloom, Chl a concentrations from the endosymbiont, P. noctilucae were around 25 mg m −3 and carbon fixation rates in excess of 2 g C m −3 day −1 at the surface and 12 g C m −2 day −1 in the 33 m euphotic column. 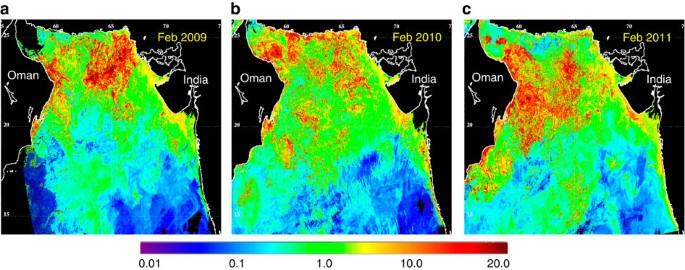Figure 2: Winter bloom seen by NASA's Aqua-MODIS satellite. Monthly (February) Aqua-MODIS Level-3 Chlorophyllaimages (binned from level 2 images at 2 km resolution) for (a) 2009, (b) 2010 and (c) 2011 showing the spatial distribution of winter phytoplankton blooms in the Arabian Sea dominated byN. scintillans. Figure 2: Winter bloom seen by NASA's Aqua-MODIS satellite. Monthly (February) Aqua-MODIS Level-3 Chlorophyll a images (binned from level 2 images at 2 km resolution) for ( a ) 2009, ( b ) 2010 and ( c ) 2011 showing the spatial distribution of winter phytoplankton blooms in the Arabian Sea dominated by N. scintillans. Full size image Our detailed study of historic taxonomic records [19] , [20] available for the winter monsoons of 1965, 1972 and 1990 averaged over an area occupied repeatedly during our ongoing cruises (19°–23°N and 64°- 69°E, Red box in Supplementary Fig. 1 ) in the Arabian Sea, show no indication of N. scintillans as a component of the winter phytoplankton community ( Fig. 3a ). Instead, diatoms were the dominant bloom-forming group ( Fig. 3a ) fuelled by the influx of nutrients into the euphotic column from winter convective mixing [3] . Similarly, taxonomic data from more contemporary, winter monsoonal expeditions such as the British ARABESQUE programme in 1994 (ref. 21 ), the U.S. JGOFS Expeditions [1] from 1994 to 1996 and the Indian JGOFS effort [22] in 1995 (also data from Red Box in Supplementary Fig. 1 ), also do not cite N. scintillans as a component of the winter phytoplankton community, but instead show diatom dominance in the offshore Arabian Sea ( Fig. 3a ). 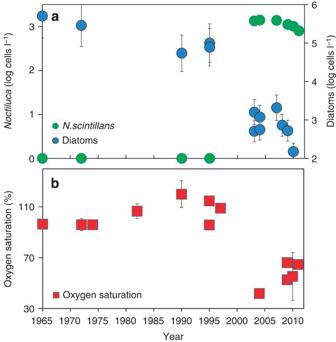Figure 3: Counts ofN. scintillansand diatoms and % seawater O2saturation. (a) Appearance ofN. scintillansin the early 2000s is associated with a concomitant decrease in total number of diatoms. Values are log of cell numbers l−1(N=3–20) averaged over red box (19°–23°N and 64°–69°E) and for cruises shown inSupplementary Fig. 1. Bars represent 10% s.e. (b) Percent O2saturation of seawater for the upper 40 m from data averaged over same red box (N=3–17) shows a decrease after 2000 whenN. scintillansblooms began appearing. In addition, vertical transects of percent O2saturation in the red box for cruises from 1974 to 2011 are shown inSupplementary Fig. 2a–f. Figure 3: Counts of N. scintillans and diatoms and % seawater O 2 saturation. ( a ) Appearance of N. scintillans in the early 2000s is associated with a concomitant decrease in total number of diatoms. Values are log of cell numbers l −1 ( N =3–20) averaged over red box (19°–23°N and 64°–69°E) and for cruises shown in Supplementary Fig. 1 . Bars represent 10% s.e. ( b ) Percent O 2 saturation of seawater for the upper 40 m from data averaged over same red box ( N =3–17) shows a decrease after 2000 when N. scintillans blooms began appearing. In addition, vertical transects of percent O 2 saturation in the red box for cruises from 1974 to 2011 are shown in Supplementary Fig. 2a–f . Full size image Our recent and detailed data on the distribution of phytoplankton species shows that the switchover from diatoms to N. scintillans in winter occurred in the early 2000s ( Fig. 3a ). Relationship of N. scintillans blooms to hypoxia On each of our cruises, we observed N. scintillans blooms in association with seawater that was undersaturated with respect to dissolved O 2 . A compilation of dissolved O 2 concentrations calculated as % oxygen saturation (data from Red box in Supplementary Fig. 1 ) over the same time period as our taxonomic data, and averaged over the euphotic column (0–40 m) shows that the appearance of near subsurface hypoxic waters offshore during the winter monsoon is a recent phenomenon that commenced in the early 2000s ( Fig. 3b , Supplementary Fig. 2a–f ), coinciding with the appearance of N. scintillans ( Fig. 3a ). Since then, annual, winter-time dissolved O 2 concentrations in the upper euphotic column have continued to remain low raising the intriguing question, whether the recurrent emergence of N. scintillans blooms in winter is being facilitated by the influx of hypoxic waters into the euphotic zone. Carbon fixation in ambient and low oxygen concentrations On cruises conducted during the N. scintillans blooms of 2010 and 2011, we carried out seven shipboard experiments (two stations in March 2010 and five stations in March 2011) to test the premise whether hypoxic waters provided N. scintillans with a more conducive environment to grow and thrive over diatoms. This was undertaken by testing if N. scintillans with its photosynthetic endosymbionts had higher carbon fixation rates at lower O 2 concentrations as compared with other phytoplankton. For each experiment, we had triplicate bottles measuring carbon fixation rates in the light and duplicate bottles to measure any dark fixation and artifacts. In six of the seven experiments conducted on board ( Fig. 4a ) with N. scintillans containing the endosymbiont, we observe significant ( P <0.05, N =21, two-sample t -test) increases in CO 2 fixation rates (25–300%), in seawater with lowered dissolved O 2 concentrations compared with ambient dissolved O 2 controls. In contrast ( Fig. 4b ), an almost three fold decrease in CO 2 fixation rates ( P <0.05, N =15, two-sample t -test) is observed in the diatom-dominated phytoplankton fraction exclusive of N. scintillans cells under the same lowered O 2 conditions. 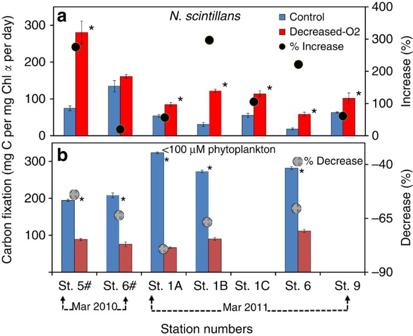Figure 4: CO2fixation by endosymbionts and <100 μM cells in decreased and ambient O2. (a) Carbon fixation rates per unit Chla(mg C per mg Chlaper day) of endosymbiontsPedinomonas noctilucaein decreased (3.0–3.2 ml l−1) versus ambient (4.75–5.0 ml l−1) concentrations of O2showed an increase in photosynthetic rates at lower dissolved O2concentrations (P<0.05,N=21, two-samplet-test). (b) Conversely, carbon fixation rates in the <100 μM fraction from whichN. scintillanshad been removed and was predominated by diatoms, decreased under lowered dissolved O2concentrations (P<0.05,N=15, two-samplet-test). Each symbol represents the average of triplicates and its s.d. % Increase/decrease is shown with black/hatched circles. All statistically significant levels (P<0.05) forPvalues obtained using two-samplet-test are denoted by *. Figure 4: CO 2 fixation by endosymbionts and <100 μM cells in decreased and ambient O 2 . ( a ) Carbon fixation rates per unit Chl a (mg C per mg Chl a per day) of endosymbionts Pedinomonas noctilucae in decreased (3.0–3.2 ml l −1 ) versus ambient (4.75–5.0 ml l −1 ) concentrations of O 2 showed an increase in photosynthetic rates at lower dissolved O 2 concentrations ( P <0.05, N =21, two-sample t -test). ( b ) Conversely, carbon fixation rates in the <100 μM fraction from which N. scintillans had been removed and was predominated by diatoms, decreased under lowered dissolved O 2 concentrations ( P <0.05, N =15, two-sample t -test). Each symbol represents the average of triplicates and its s.d. % Increase/decrease is shown with black/hatched circles. All statistically significant levels ( P <0.05) for P values obtained using two-sample t -test are denoted by *. Full size image Autotrophic and phagotrophic feeding in N. scintillans In addition to establishing that carbon fixation rates of N. scintillans were higher in waters with lowered dissolved O 2 , we also conducted shipboard experiments to elucidate the interplay between the dependence of N. scintillans on its autotrophic endosymbionts, and its facultative phagotrophy of associated phytoplankton during the bloom ( Fig. 5 ). Results indicate that when N. scintillans is grown in the dark with or without food, its growth rates are much lower ( P <0.001, two-sample t -test, P and N values in Supplementary Table 1 ) than in the light, indicating the importance of the autotrophic endosymbionts for growth. When nutrients are added to the ‘No Food’ set of bottles, growth rates are significantly enhanced over controls ( P <0.01, two-sample t -test, P and N values in Supplementary Table 1 ) reinforcing the view that N. scintillans can meet its metabolic needs via its autotrophic endosymbionts. If, however, extraneous food and light are available, growth rates of N. scintillans are comparable to treatments with only nutrients and light ( P <0.721, two-sample t -test, P and N values in Supplementary Table 1 ) indicating that N. scintillans can also sustain its growth via phagotrophy. The lack of any further increase in growth rates, when nutrients are added to flasks containing food and exposed to light, suggests that when food is available, N. scintillans is capable of meeting a large fraction of its metabolic requirements via phagotrophy. Conversely, when food becomes scarce but nutrients are available, N. scintillans meets its metabolic needs via carbon fixation by its autotrophic endosymbionts. A comparison of growth rates of N. scintillans grown in the dark with and without food shows that starved cells had higher growth rates than cells which were provided with food. One reason for this may be that the lack of light caused the food (mainly phytoplankton) to die and decay, increasing bacterial respiration and lowering oxygen. 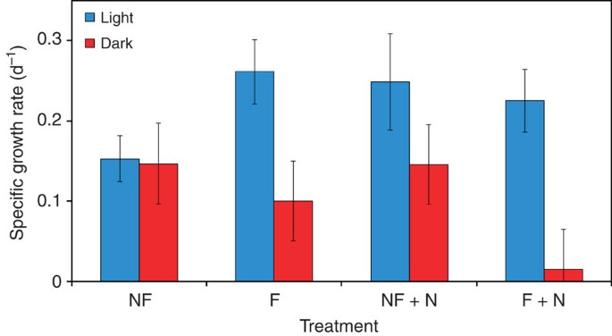Figure 5: Growth rates ofN. scintillanswith and without food, light and nutrients. Specific growth rates ofN. scintillansincubated for 96 h with food (F) and without food (NF), with or without nutrients (N) and in light and dark condition to assess the relative importance of internal nutrition from symbionts and external phagotrophy for growth ofN. scintillans. Addition of f/50 nutrients (N) was meant to support endosymbiotic photosynthesis. For incubations without added nutrients bars represent mean±one s.d. for three replicate incubations. For incubations with nutrients, bars represent means±one s.d. for eight replicate incubations. Statistically significant levels forPvalues obtained using two-samplet-test are shown inSupplementary Table 1. Figure 5: Growth rates of N. scintillans with and without food, light and nutrients. Specific growth rates of N. scintillans incubated for 96 h with food (F) and without food (NF), with or without nutrients (N) and in light and dark condition to assess the relative importance of internal nutrition from symbionts and external phagotrophy for growth of N. scintillans . Addition of f/50 nutrients (N) was meant to support endosymbiotic photosynthesis. For incubations without added nutrients bars represent mean±one s.d. for three replicate incubations. For incubations with nutrients, bars represent means±one s.d. for eight replicate incubations. Statistically significant levels for P values obtained using two-sample t -test are shown in Supplementary Table 1 . Full size image Impact of N. scintillans blooms on the food web Recognizing that its large size can preclude it from being grazed on by conventional grazers of phytoplankton [23] , we conducted preliminary experiments to assess the potential of N. scintillans as a food source. During all cruises, N. scintillans blooms were observed in association with large population of salps. In 2011, we conducted grazing experiments on board that estimated clearance rates of 200 to 800 ml per hour for the salp Pegea confoederata , suggesting that high concentrations of salps (up to hundreds of zooids per m 2 ) could rapidly consume dense aggregations of N. scintillans . Using pigments [7] , [24] as a measure of food consumed in the first 3 h, we observed that single salps can remove on average 71% of Chl a and 78% of Chl b from seawater dominated by N. scintillans cells with the deposition of large pellets ( Supplementary Fig. 3a ). Our results show that the advent of N. scintillans during the winter monsoon is tied to a recent decrease in dissolved O 2 content of the upper water column of the Arabian Sea. Favourable growth of N. scintillans under hypoxia is not unrealistic, given that its endosymbiont P. noctilucae evolved 1.3 Ga years ago when oceanic O 2 concentrations were much lower than in the modern world, making its carbon assimilation pathways and enzyme systems more uniquely suited to hypoxic environments [25] . Oxygen deficiency [26] , [27] in the northeastern Arabian Sea is a unique mid-depth (>120–1,500 m) feature formed by the combined influences of monsoon-driven high surface productivity of the semi-annual phytoplankton blooms, sub-thermocline source waters that have naturally low dissolved O 2 content flowing from the Southern Ocean and poor ventilation of subsurface waters in the landlocked north. Except for summer coastal upwelling that is known to bring up hypoxic waters on to the western Indian shelf [13] , there are no known physical mechanisms to explain the appearance of O 2 deficient waters above 40 m in the offshore region in winter. The possibility that intensification of winter-time penetrative mixing is causing an influx of deeper (>150 m) O 2 poor water into subsurface waters had to be ruled out as the Arabian Sea appears to be experiencing a shallowing of Mixed Layer ( Supplementary Fig. 4a,b ), a feature consistent with a weakening of winter convective mixing. Another possibility is that the Arabian Sea’s permanent oxygen minimum zone is expanding horizontally and vertically because of increased organic matter delivery to deeper depths, a notion supported by our recent findings [28] that the Arabian Sea is becoming more productive due to warming of the Eurasian continent and the systematic decrease in spring snow persistence over large parts of southwest Asia and the Himalayan–Tibetan Plateau region. Loss of snow persistence in recent years has enhanced the land–sea pressure gradient, which in turn has strengthened southwest monsoonal winds resulting in intensified wind-driven coastal upwelling favoring enhanced phytoplankton blooms during summer. Another potential source of organic matter to the Arabian Sea is domestic and industrial outfall from countries bordering the Arabian Sea. One such region is the western shelf of the Indian subcontinent, where waste water treatment plants have not kept pace with rapid population growth and urbanization of coastal cities [29] , [30] . The population of Metropolitan Mumbai Region alone has doubled over the last decade to 21 million and discharges 2,700 megaliters per day of severely O 2 -depleted (0–2.85 ml l −1 ), nutrient-rich (7–35 μM of NO 3 , 0.3–25 μM of PO 4 , 0.8–24 μM of NH 3 ) domestic waste water containing 63 tons of nitrogen and 11 tons of phosphorous into the eastern Arabian Sea [31] . To the north, Karachi whose current population is 15 million discharges about 1,600 megaliters per day of domestic and industrial waste water of which 70% is untreated, severely O 2 -depleted and nutrient and organic material-rich [32] . Dissolved O 2 concentrations available from the Government of India’s Ministry of Earth Sciences long-term monitoring programme called Coastal Ocean Monitoring and Prediction System are generally very low (1.4±1.23 ml l −1 ) in winter. We hypothesize that during winter, the poleward flowing West Indian Coastal Current [33] ( Supplementary Fig. 1 ) may be facilitating the spread of hypoxic waters offshore. The terrestrial origin of these hypoxic waters during winter is evident from the warm, low salinity, low density characteristics of these waters seen along almost the entire eastern boundary of the Arabian Sea ( Supplementary Fig. 5a–e ). In addition, plots of dissolved O 2 data along density isopycnals ( Fig. 6a–c ) also provide indications of the coastal origins of surface hypoxia. Data from the 1980s and 1990s for instance show hypoxia associated with colder and denser waters from depth ( Fig. 6a,b ) in contrast to observations of the 2000s, which show hypoxia at much shallower depths associated with warm, low salinity and low density waters indicating their coastal origins ( Fig. 6c ). 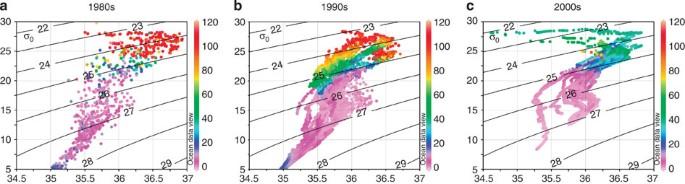Figure 6: Temperature–Salinity plots showing major water masses and O2(ml l−1). (a) O2concentrations represented by the color of the data points show hypoxic conditions in colder and denser waters at depth in the 1980s. (b) Gradual shoaling of O2deficient waters into the subsurface waters in the 1990s. (c) Appearance of hypoxic waters at the surface in the 2000s. High temperature, low salinity and low density signatures of these waters reveal their terrestrial influence. Figure 6: Temperature–Salinity plots showing major water masses and O 2 (ml l −1 ). ( a ) O 2 concentrations represented by the color of the data points show hypoxic conditions in colder and denser waters at depth in the 1980s. ( b ) Gradual shoaling of O 2 deficient waters into the subsurface waters in the 1990s. ( c ) Appearance of hypoxic waters at the surface in the 2000s. High temperature, low salinity and low density signatures of these waters reveal their terrestrial influence. Full size image Shoaling of O 2 -depleted waters has been observed very frequently on the continental shelf of the west coast of India, but always in summer, due to coastal upwelling. Earlier reports [34] have shown an intensification of O 2 depletion in these freshly upwelled waters with possible links to increased agricultural fertilizer usage in this region but, the recent albeit few available data from Indian estuarine studies [16] , [35] are not supportive of such high nutrient loading. However, considering the explosive growth in the use of synthetic fertilizers in South Asia over the last 1.5 decades, the consumption of which in 2012 alone was estimated at 17.5 million metric tonnes of urea and 15 million metric tonnes of ammonia [36] , it is not unreasonable to expect the Arabian Sea could also be witnessing the long-term impacts of excessive fertilizer usage, similar to other coastal ecosystems experiencing hypoxia. Another potential source of new nitrogen into the Arabian Sea is atmospheric deposition, but recent estimates show that it contributes only about 3% to new production in the Arabian Sea [37] . The emergence of N. scintillans as the dominant bloom-forming organism in the northern Arabian Sea requires careful evaluation of its role in the food web. N. scintillans does not appear to be a preferred food source for common mesozooplankton, in part because it is too large to be grazed ( Supplementary Fig. 3b ) especially by copepods, the most common grazers of diatoms [23] , that used to proliferate in the winter bloom. Instead its most notable consumers are jellyfish and salps ( Supplementary Fig. 3c–e ). Thus, in addition to causing a shift in planktonic communities from dominance by diatoms and copepods at the lower trophic level, N. scintillans can alter trophic interactions via carbon transfer to salps and jellyfish, both minor components of fish diet. Although laboratory strains of N. scintillans can survive for more than 2 years solely on their endosymbionts [38] , in natural conditions their growth to bloom proportions appears to be aided by the presence of a large population of diatoms, which are visible in their food vacuoles ( Fig. 1b , Supplementary Fig. 3f ). While the ability of the endosymbionts to fix carbon more efficiently than diatoms under hypoxic conditions can allow N. scintillans to outgrow diatoms, increased nutrients from winter convective mixing, abundant light and the ability of N. scintillans to feed on diatoms, allow it to proliferate for almost 2 months, contributing to the overall loss of diatoms witnessed in recent years. The traditional 14 C method [39] of measuring carbon fixation on oceanographic cruises employed in this study does not allow us to elucidate the mechanism that enhances carbon fixation in the endosymbiont of N. scintillans at low ambient O 2 concentrations, nor does it help explain why carbon fixation rates were reduced in diatoms. We hope that our future planned studies involving transcriptome level analysis of phytoplankton responding to ambient O 2 conditions, both in field and in culture, will help us better understand these complex photosynthetic carbon assimilation mechanisms in different phytoplankton. On its own, N. scintillans does not appear to contribute significantly to particulate organic carbon export judging from the absence of any cells in shallow water sediment traps deployed during our cruises. Instead, the major delivery of carbon into the deep appears to be largely in the form of large and rapidly sinking faecal pellets ( Supplementary Fig. 3a ) from salps and jellyfish. The magnitude of this flux together with more robust measurements of carbon fixation and export rates mediated by N. scintillans blooms, as well as estimates of the anthropogenic loading of organic matter from coastal megacities need to be carefully assessed since any further increases in carbon flux could make the region even more susceptible to hypoxia and N. scintillans blooms to the detriment of regional fisheries. Significant deoxygenation of seawater has been reported over the past 50 years in tropical oceans [40] , [41] . Ocean models [42] predict declines of 1 to 7% in the global ocean O 2 inventory over the next century due to global warming, water column stratification, rising atmospheric CO 2 and enhanced nutrient inputs, the latter attributable to continued fertilizer usage and the growth of coastal cities as well as from continental dust storms. Evidence of significant impacts on marine biota has raised the spectre of imminent impacts on marine habitats and fisheries, but these observations have come largely from coastal ecosystems experiencing repeated assaults of severely oxygen-depleted waters. What makes the Arabian Sea unique and a special cause for concern is that changes in its biota are occurring offshore and on a basin-wide scale. Seawater sample collection On all cruises conducted from 2003 to 2011, seawater samples were collected with a 5-L Niskin sampler mounted on a Sea Bird Electronics CTD Rosette using prescribed clean techniques [39] . Measurement of physical and chemical parameters Calibrated sensors on the CTD provided vertical profiles of salinity, temperature and dissolved O 2 . The salinity sensor was calibrated against Autosal Salinometer measurements, while the dissolved O 2 sensor was calibrated against measurements using the Winkler and colorimetric-end point automated titration procedures [39] in seawater samples from discrete depths. From 2009 onwards, dissolved O 2 was measured exclusively by the Winkler method with high-precision amperometric end point detection [43] . Dissolved O 2 concentrations from April 1989 to April 2007 off the coast of Mumbai are from the Government of India’s Ministry of Earth Sciences long-term monitoring programme, Coastal Ocean Monitoring and Prediction System. For this set of data, dissolved O 2 concentrations (ml l −1 ) were measured using the Winkler and colorimetric-end point automated titration procedures [39] . Historic dissolved O 2 data Historic dissolved O 2 data was obtained from the Data Center of the National Institute of Oceanography, Goa, India. Quality control was guided by the National Oceanographic Data Center Report and included duplicate profile, depth duplication, data range and large temperature and inversion checks [44] . % O 2 saturation was calculated using Ocean Data View with inputs of concomitant measurements of dissolved O 2 (μm kg −1 ), temperature, salinity and depth. Mixed layer depths Mixed layer depth was computed based on the 1 °C gradient from the surface using temperature data from GODAS. Relative humidity was derived from NCEP-NCAR reanalysis monthly products from ( http://www.cpc.ncep.noaa.gov/products/GODAS/ ). Source for coastal population statistics Coastal population quoted in the abstract is from the NASA Socioeconomic Data and Applications Centre, Centre for International Earth Science Information Network, Columbia University, New York, USA. ( http://sedac.ciesin.columbia.edu/gpw ) Historical and current phytoplankton taxonomical analysis Microscopic identification and enumeration of phytoplankton were undertaken on duplicate samples fixed with 1% Lugol’s iodine in 3% buffered formaldehyde solution and stored in cool and dark conditions for cells to settle. Before microscopy, samples were concentrated to 5–10 ml by siphoning out the top layer through a 10 μm Nitex filter wrapped around the tip of a thin tube. Although microscopic examination of the siphoned layer indicated that no visible cells, cell abundance estimated using this method only applies to >10 μm cells. One ml replicates of the concentrated sample were transferred on to a Sedgwick-Rafter slide and cell numbers were enumerated with an Olympus Inverted microscope (Model IX 50) at × 200 magnification. Identification of phytoplankton was based on standard taxonomic keys [45] , and was in most cases undertaken up to the species level. Historic phytoplankton data was downloaded from Open Access library PANGAEA. Samples were concentrated by gravity filtration. Samples from February to March 1965, 1972 and March 1995 were preserved in Lugol’s iodine while in February 1990 they were counted live on board the ship. Oxygen experiments Carbon fixation rates of carefully separated N. scintillans cells and of the <200 μm fraction without N. scintillans cells, were measured under decreased O 2 and ambient (control) conditions using the modified radioactive NaH 14 CO 3 tracer technique where the uptake of the tracer is estimated based on its transformation to particulate organic form [39] . Experiments were performed at two stations in March 2010 and five stations in March 2011 during the bloom. For each experiment, seawater containing N. scintillans was collected from the surface with a Niskin sampler approximately 3 h before sunrise. Before isolation of the N. scintillans cells, 26, 125 ml stoppered glass bottles were filled with 0.22 μm Nucleopore filtered seawater (FSW) from the same location to remove all cells and detrital particles. Dissolved O 2 in one set of 13 bottles was reduced to ~25% of its original concentration by gently purging the FSW in the bottles with a mixture of high purity N 2 and CO 2 (375 p.p.m.) gases. The dissolved O 2 in the other set of 13 bottles was left unpurged and served as controls. Initial dissolved O 2 concentrations in three bottles each from the purged and from the control sets were measured using the Winkler method with high-precision amperometric end point detection [43] . Average dissolved O 2 in purged and control sets was 3.0–3.2 ml l −1 and 4.75–5.0 ml l −1 respectively. The remaining 20 bottles (10 purged and 10 controls) were used to measure the carbon fixation rates of N. scintillans cells and of the <200 μm phytoplankton in low and ambient oxygen concentrations of seawater. N. scintillans cells were isolated by gently filtering seawater through a 200-μm mesh net placed in a beaker containing FSW to provide buffering for cells. Individual N. scintillans cells were carefully picked with a glass Pasteur pipette and transferred to another beaker containing FSW to make an evenly distributed cell concentrate. Two ml aliquots of the concentrate were carefully added to five purged and five control bottles with minimal exposure to atmospheric O 2 . In addition, 2 ml aliquots of the concentrate were filtered in triplicate onto GF/F filters, frozen in liquid nitrogen and transported to the shore for estimation of biomass as Chl a by high-performance liquid chromatography (HPLC) [7] , [24] . One ml of a 5 μCi of NaH 14 CO 3 solution was added to the 10 bottles of purged and control sets containing N. scintillans . Three of the five bottles were incubated in light to estimate autotrophic 14 C fixation in triplicate and two were incubated in dark to correct for dark uptake of CO 2 and abiotic formation of labelled particulate carbon. Dark bottles were covered with double-layered cloth bags with Velcro closures. The remaining five purged and five control bottles were used to measure carbon fixation [39] of the <200 μm fraction of phytoplankton, devoid of N. scintillans and comprising mainly of diatoms. The filtrate collected after removing N. scintillans cells, was concentrated by gently passing through a 10-μm mesh net and immediately resuspended in FSW. Microscopic examination showed the suspension to contain predominately diatoms (70–94%) and dinoflagellates. Two ml of this concentrate was added to each of the 10 bottles containing FSW, followed by the NaH 14 CO 3 solution. Samples were also collected for estimation of the biomass (as Chl a ) of the <200 μm fraction by HPLC [7] , [24] . All bottles were incubated on deck (at ~30% of ambient direct sunlight using neutral density screening, measured with a LI-190 Quantum sensor) in running seawater to approximate in situ conditions. The incubation bottles were removed after exactly 24 h, filtered through 0.45 μM Millipore membrane filters which were then fumed with HCl to remove any excess inorganic NaH 14 CO 3 adsorbed on the filters. Activity was measured with a Perkin Elmer Liquid Scintillation Counter and DPM values were converted to daily productivity rates [39] (mg C m −3 day −1 ) after subtracting the average dark bottle DPM from average DPM of three light bottles (triplicate). Autotrophy versus phagotrophy experiments Measurements of the growth rates of N. scintillans were made separately in deck incubators (conditions described above) for 96 h to assess the relative importance of internal nutrition from endosymbionts and external phagotrophy for growth of N. scintillans . Groups of 10 cells of N. scintillans were incubated in 70 ml Corning tissue culture flasks under reduced sunlight (see above) or in darkness (flask wrapped in aluminium foil) in either 0.45 μm Nybolt membrane FSW (no food), or whole seawater with natural plankton assemblage increased to five times the normal concentration (food) by gentle reverse filtration through a 20-μm mesh. Ambient nutrient concentrations in these experiments ranged from 0.37 to 0.66 μM for inorganic nitrate, 0.20 to 0.38 μM for inorganic phosphate and from 1.99 to 5.09 μM for silicate. Another set of experiments with N. scintillans from the same bloom were performed in which nutrient concentrations within the tissue culture flasks were enhanced with 17.6 μM inorganic nitrate and 0.7 μM inorganic phosphate. At the end of the incubation period, cell cells were counted using an Olympus SZX10 stereomicroscope. Specific growth rates (μ d −1 ) were calculated as the natural logarithm of the number of cells present at the end of the experiment minus the natural logarithm of the number of cells at the beginning of the experiment divided by the duration of the experiment in days. Although N. scintillans is capable of cannibalism, which could compromise growth rate estimates, it is mainly a problem when N. scintillans densities are high and food is scarce. Our experiments had only 10 cells per culture flask. In addition, we observed the light treatments with and without food daily and found no increase in N. scintillans numbers followed by a decline as would be expected if initial growth followed by cannibalism after starvation or food depletion occurred. Salp grazing experiments Clean 10 l buckets were used to collect surface N. scintillans bloom populations. Triplicate samples of 50 ml were filtered onto GF/F glass fibre filters and immediately transferred into a liquid nitrogen Dewar for HPLC [7] , [24] measurements of pigment concentrations at Time zero. Live salps were collected separately from which single adult salps were carefully picked, transferred into FSW for about 2 h to empty their guts and then into the buckets containing the N. scintillans bloom. After a 4-h incubation period when the buckets were incubated in running seawater in the dark, 50 ml samples were collected in triplicate for post incubation pigment analysis by HPLC [7] , [24] . In addition, the faecal pellets that were formed were carefully picked and placed in petri dishes. How to cite this article: Gomes, H. do R. et al. Massive outbreaks of Noctiluca scintillans blooms in the Arabian Sea due to spread of hypoxia. Nat. Commun. 5:4862 doi: 10.1038/ncomms5862 (2014).